The TSC-mTOR pathway regulates macrophage polarization Macrophages are able to polarize to proinflammatory M1 or alternative M2 states with distinct phenotypes and physiological functions. How metabolic status regulates macrophage polarization remains not well understood, and here we examine the role of mTOR (mechanistic target of rapamycin), a central metabolic pathway that couples nutrient sensing to regulation of metabolic processes. Using a mouse model in which myeloid lineage-specific deletion of Tsc1 ( Tsc1 Δ/Δ ) leads to constitutive mTOR complex 1 (mTORC1) activation, we find that Tsc1 Δ/Δ macrophages are refractory to IL-4-induced M2 polarization, but produce increased inflammatory responses to proinflammatory stimuli. Moreover, mTORC1-mediated downregulation of Akt signalling critically contributes to defective polarization. These findings highlight a key role for the mTOR pathway in regulating macrophage polarization, and suggest how nutrient sensing and metabolic status could be ‘hard-wired’ to control of macrophage function, with broad implications for regulation of type 2 immunity, inflammation and allergy. Macrophages have a dynamic role in host defense and maintenance of tissue homoeostasis. This necessitates a delicate balance between their proinflammatory and immunomodulatory functions to ensure appropriate responses to environmental stimuli. Macrophages can be broadly classified into M1 (classical) and M2 (alternative) subtypes based on function. M1 macrophages are activated by LPS and/or IFN-γ to elaborate proinflammatory cytokine production and tissue inflammation [1] . Conversely, M2 macrophages are stimulated by Th2 cytokines IL-4 and/or IL-13 to promote helminthic immunity, fibrosis, allergy and immunomodulation [2] . Stimulation of macrophages with IL-4 and IL-13 leads to activation of the transcription factor STAT6, which is indispensable for M2 polarization [3] . In addition, activation of the nuclear receptors PPARγ and PPARδ is necessary for full implementation of the M2 programme [4] , [5] . A hallmark of M2 macrophages is an increase in Arginase-1 gene expression and activity [2] , which converts L -arginine to L -ornithine to promote polyamine synthesis and tissue repair [6] . The M2 programme is also characterized by upregulation of C-type lectins, mannose receptor, chitinase family proteins, resistin-like molecules and Interleukin-10, all of which contribute to immunomodulatory function [7] . Importantly, distinct metabolic programs are required to support energy demands of M1 and M2 macrophages. M1 macrophages rely primarily on glycolytic metabolism, mediated by HIF-1α, whereas M2 macrophages utilize fatty acid oxidation mediated by PPARγ and the transcriptional coactivator, PGC-1β (refs 3 , 8 , 9 ). This suggests that macrophage metabolism and inflammatory phenotype are integrally linked, and hint at additional regulatory control of macrophage polarization by metabolic pathways. The mechanistic target of rapamycin (mTOR) is a key nutrient/energy sensor that couples nutrient availability to regulation of downstream metabolic processes such as protein synthesis, glycolysis and de novo lipogenesis [10] , [11] . mTOR, a serine/threonine kinase, exists in a rapamycin-sensitive complex called mTORC1 that is negatively regulated by the tuberous sclerosis complex comprising TSC1 and TSC2 (ref. 12 ). Genetic loss of either TSC1 or TSC2 leads to constitutive mTORC1 activation [13] . Importantly, recent studies demonstrate that mTOR controls multiple aspects of T-cell biology including quiescence, activation and differentiation [14] . However, little is known regarding the role of mTOR in regulating macrophage activation. In the current study, we elucidate a role for mTOR in macrophage polarization. We demonstrate that Tsc1 Δ/Δ macrophages have a marked defect in M2 polarization in response to IL-4, whereas the inflammatory response to LPS is enhanced. Aberrant polarization is due, at least in part, to mTORC1-mediated attenuation of Akt activity, which renders Tsc1 Δ/Δ macrophages resistant to the immunomodulatory effects of Akt downstream of IL-4 and LPS signalling. Finally, we show that IL-4 and chitin administration in Tsc1 Δ/Δ mice recapitulates the defective M2 polarization in vivo. Constitutive mTORC1 activity impairs M2 polarization The mTOR pathway integrates a variety of inputs to regulate cell growth and to balance anabolic and catabolic processes [15] . Interestingly, stimulation of bone marrow-derived macrophages (BMDMs) with IL-4 or LPS resulted in mTORC1 activation as indicated by increased phosphorylation of the downstream targets S6K1 and 4E-BP1 ( Fig. 1a ), suggesting that the mTORC1 pathway may coordinate metabolic changes during macrophage activation. To examine this hypothesis, we utilized a model of myeloid-specific Tsc1 deficiency in which mTORC1 is constitutively active. Tsc1 loxP/loxP LysMCre mice and Tsc1 loxP/loxP controls are herein referred to as Tsc1 Δ/Δ and Tsc1 fl/fl , respectively. Immunoblotting confirmed that TSC1 is absent in the Tsc1 Δ/Δ BMDMs ( Fig. 1b ). TSC2 protein level was also diminished ( Fig. 1b ), as TSC1 stabilizes TSC2 (ref 16 ). Tsc1 Δ/Δ BMDMs displayed constitutive phosphorylation of the mTORC1 downstream targets S6K1 and 4E-BP1, as well as the S6K1 target ribosomal S6, all of which were sensitive to the mTORC1-specific inhibitor, rapamycin ( Fig. 1b ). Furthermore, Tsc1 Δ/Δ BMDMs seemed to differentiate normally in vitro and expressed similar levels of the macrophage markers F4/80 and CD11b ( Supplementary Fig. S1 ). As reported in other models of TSC deficiency [17] , Tsc1 Δ/Δ BMDMs were larger ( Supplementary Fig. S1 ) due likely to a role of mTORC1 in regulating cell size [18] . These observations confirmed constitutive mTORC1 activation in Tsc1 Δ/Δ BMDMs and established the validity of our genetic model. 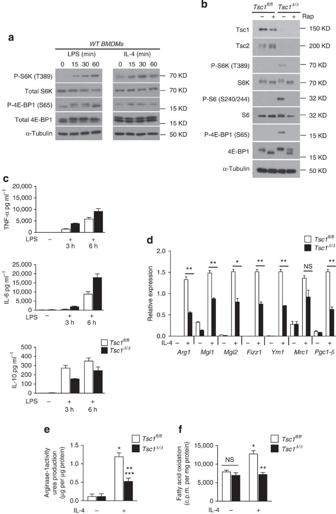Figure 1:Tsc1Δ/ΔBMDMs have defective M2 polarization and enhanced responses to LPS stimulation. (a) Immunoblot analysis of WT BMDMs stimulated with LPS or IL-4 for 15–60 min as indicated. (b) Immunoblot analysis of lysates fromTsc1fl/flandTsc1Δ/ΔBMDMs treated with or without rapamycin for 15 h. (c) Measurement of TNF-α, IL-6 and IL-10 secretion by ELISA after treatment with LPS for 3 h and 6 h, (n=2 representative experiments). (d) Expression of M2 genes inTsc1fl/flandTsc1Δ/ΔBMDMs after treatment with IL-4 for 24 h (n=3). *P<0.05, **P<0.01, ***P<0.001. (e) Urea production normalized to total protein inTsc1fl/flandTsc1Δ/ΔBMDMs stimulated as in (c), (n=4) *P<0.001 for untreated versus IL-4 forTsc1fl/fl, **P<0.01 for IL-4 treatedTsc1fl/flversusTsc1Δ/Δ, ***P<0.05 for untreated versus IL-4 forTsc1Δ/Δ. (f) Fatty acid oxidation of3H-palmitic acid presented as counts per minute normalized to milligram of total protein after 36 h treatment with IL-4, (n=3). *P<0.01 for untreated versus IL-4 inTsc1fl/fl, **P<0.01 for IL-4 treatedTsc1fl/flversusTsc1Δ/Δ. Graphs are shown as mean±s.e.m.Pvalues were determined using Student’st-tests. Figure 1: Tsc1 Δ/Δ BMDMs have defective M2 polarization and enhanced responses to LPS stimulation. ( a ) Immunoblot analysis of WT BMDMs stimulated with LPS or IL-4 for 15–60 min as indicated. ( b ) Immunoblot analysis of lysates from Tsc1 fl/fl and Tsc1 Δ/Δ BMDMs treated with or without rapamycin for 15 h. ( c ) Measurement of TNF-α, IL-6 and IL-10 secretion by ELISA after treatment with LPS for 3 h and 6 h, ( n =2 representative experiments). ( d ) Expression of M2 genes in Tsc1 fl/fl and Tsc1 Δ/Δ BMDMs after treatment with IL-4 for 24 h ( n =3). * P <0.05, ** P <0.01, *** P <0.001. ( e ) Urea production normalized to total protein in Tsc1 fl/fl and Tsc1 Δ/Δ BMDMs stimulated as in ( c ), ( n =4) * P <0.001 for untreated versus IL-4 for Tsc1 fl/fl , ** P <0.01 for IL-4 treated Tsc1 fl/fl versus Tsc1 Δ/Δ , *** P <0.05 for untreated versus IL-4 for Tsc1 Δ/Δ . ( f ) Fatty acid oxidation of 3 H-palmitic acid presented as counts per minute normalized to milligram of total protein after 36 h treatment with IL-4, ( n =3). * P <0.01 for untreated versus IL-4 in Tsc1 fl/fl , ** P <0.01 for IL-4 treated Tsc1 fl/fl versus Tsc1 Δ/Δ . Graphs are shown as mean±s.e.m. P values were determined using Student’s t -tests. Full size image To assess macrophage polarization in Tsc1 Δ/Δ BMDMs, we used LPS treatment to promote an M1-like phenotype and IL-4 stimulation to induce an M2 phenotype. We found that LPS-treated Tsc1 Δ/Δ BMDMs secreted more of the proinflammatory cytokines IL-6 and TNF-α, but less of the anti-inflammatory cytokine IL-10 ( Fig. 1c ). Given the enhanced responses of Tsc1 Δ/Δ BMDMs to LPS, we postulated that M2 polarization could be defective. Indeed, Tsc1 Δ/Δ BMDMs failed to fully upregulate the M2 programme, with significant reductions in Arg1 , Mgl1 , Mgl2 , Ym1 , Fizz1 and Pgc1-β expression ( Fig. 1d ). Arginase-1 activity assessed by urea production was reduced, correlating with lower levels of Arg1 messenger RNA ( Fig. 1e ). IL-4-stimulated fatty acid oxidation, another hallmark feature of M2 macrophages, was also defective ( Fig. 1f ). This finding is consistent with the threefold reduction in Pgc1-β ( Fig. 1d ), a known mediator of fatty acid oxidation in M2 macrophages [9] . Interestingly, M2c polarization triggered by IL-10 stimulation was also deficient in Tsc1 Δ/Δ BMDMs ( Supplementary Fig. S2a ), which may indicate impaired orchestration of anti-inflammatory responses during tissue remodelling or wound healing [19] . Macrophage activation to the M2b phenotype (by treatment with LPS/immune complexes), which has features of both M1 and M2 macrophages [20] , [21] , was not affected ( Supplementary Fig. S2b ). Taken together, our findings demonstrate that aberrant mTORC1 activation critically modulates macrophage polarization. Impaired induction of Pgc-1β and fatty acid oxidation also highlights a key role of mTOR in orchestrating macrophage cellular metabolism. STAT6 and PPARγ activity are normal in Tsc1 Δ/Δ BMDMs IL-4R signalling leads to activation of JAK1/JAK3 and tyrosine phosphorylation of the transcription factor STAT6, enabling nuclear translocation [2] and induction of target genes such as Pparγ and Arg1 (ref. 3 ). To interrogate the mechanism underpinning defective M2 polarization in Tsc1 Δ/Δ BMDMs, we first examined signal transduction downstream of the IL-4R. Tsc1 Δ/Δ BMDMs expressed comparable levels of Jak1 , Jak3 and IL-4rα messenger RNA as well as STAT6 protein at basal state ( Fig. 2a , Supplementary Fig. S3a ). Following IL-4 stimulation, STAT6 was tyrosine phosphorylated consistent with normal activation ( Fig. 2a ). Chromatin immunoprecipitation assays indicated comparable IL-4-induced recruitment of STAT6 to the promoter of the Arg1 gene ( Supplementary Fig. S3b ). Furthermore, IL-4-inducible STAT6 transcriptional activity as measured by a STAT6 reporter assay was unaffected ( Fig. 2b ). Finally, normal induction of some M2 genes in Tsc1 Δ/Δ BMDMs, including the STAT6-dependent gene Ppar γ [22] ( Fig. 2c ), indicates no general defect in the expression or activation of STAT6, the master regulator of M2 gene induction. IL-4 signalling can activate STAT1 in some contexts [23] , [24] , but not in macrophages ( Supplementary Fig. S3c ) consistent with a prior report, excluding a role for impaired STAT1 activation in the phenotype of Tsc1 Δ/Δ BMDMs [25] . 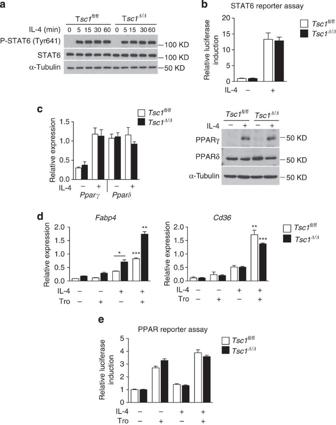Figure 2: STAT6 and PPARγ activity are normal inTsc1Δ/ΔBMDMs. (a) Immunoblot analysis of lysates fromTsc1fl/flandTsc1Δ/ΔBMDMs stimulated with IL-4 for 5–60 min. (b) STAT6 luciferase reporter assay inTsc1fl/flandTsc1Δ/ΔBMDMs. Data shown as fold induction of firefly luciferase activity normalized to renilla luciferase for IL- 4 treatment relative to untreated sample (n=2 experiments performed in duplicate). (c) Gene expression and immunoblots for PPARγ and PPARδ inTsc1fl/flandTsc1Δ/ΔBMDMs after treatment with IL-4 for 24 h. Gene expression data are shown as mean±s.e.m. (n=3). (d) Expression of PPARγ-dependent genes inTsc1fl/flandTsc1Δ/ΔBMDMs treated with IL-4 in the presence or absence of troglitazone for 24 h. DMSO vehicle was used as control,(n=3). *P<0.05 for IL-4 treatedTsc1fl/flandTsc1Δ/Δ, **P<0.01, ***P<0.001 for IL-4 versus IL-4+Tro. (e) PPAR luciferase reporter assay inTsc1fl/flandTsc1Δ/ΔBMDMs. Data shown as fold induction of firefly luciferase activity normalized to renilla luciferase for IL-4 or troglitazone treatment relative to untreated sample (representative of three experiments performed in triplicate). Graphs are shown as mean±s.e.m.Pvalues determined using Student’st-tests. Figure 2: STAT6 and PPARγ activity are normal in Tsc1 Δ/Δ BMDMs. ( a ) Immunoblot analysis of lysates from Tsc1 fl/fl and Tsc1 Δ/Δ BMDMs stimulated with IL-4 for 5–60 min. ( b ) STAT6 luciferase reporter assay in Tsc1 fl/fl and Tsc1 Δ/Δ BMDMs. Data shown as fold induction of firefly luciferase activity normalized to renilla luciferase for IL- 4 treatment relative to untreated sample ( n =2 experiments performed in duplicate). ( c ) Gene expression and immunoblots for PPARγ and PPARδ in Tsc1 fl/fl and Tsc1 Δ/Δ BMDMs after treatment with IL-4 for 24 h. Gene expression data are shown as mean±s.e.m. ( n =3). ( d ) Expression of PPARγ-dependent genes in Tsc1 fl/fl and Tsc1 Δ/Δ BMDMs treated with IL-4 in the presence or absence of troglitazone for 24 h. DMSO vehicle was used as control,( n =3). * P <0.05 for IL-4 treated Tsc1 fl/fl and Tsc1 Δ/Δ , ** P <0.01, *** P <0.001 for IL-4 versus IL-4+Tro. ( e ) PPAR luciferase reporter assay in Tsc1 fl/fl and Tsc1 Δ/Δ BMDMs. Data shown as fold induction of firefly luciferase activity normalized to renilla luciferase for IL-4 or troglitazone treatment relative to untreated sample (representative of three experiments performed in triplicate). Graphs are shown as mean±s.e.m. P values determined using Student’s t -tests. Full size image Because previous studies indicate a key role for the nuclear receptors PPARγ and PPARδ in M2 polarization, we next turned to an analysis of their expression and activity in Tsc1 Δ/Δ BMDMs. First, we showed comparable expression of PPARγ and PPARδ in Tsc1 fl/fl and Tsc1 Δ/Δ BMDMs, at basal state and after IL-4 stimulation ( Fig. 2c ). As the expression does not necessarily reflect functional activity, we examined PPARγ activity in Tsc1 Δ/Δ BMDMs. We found that IL-4-induced comparable expression of the canonical PPARγ-dependent genes Fabp4 (refs 22 , 26 ) and Cd36 (ref. 27 ) ( Fig. 2d ). Furthermore, the PPARγ agonist troglitazone synergized with IL-4 to a similar extent in Tsc1 fl/fl and Tsc1 Δ/Δ BMDMs ( Fig. 2d ). Analogous findings were obtained with the PPARδ-dependent gene Atgl [28] using the PPARδ agonist GW501516 ( Supplementary Fig. S4 ). To corroborate gene expression data, we used a PPAR reporter assay to assess PPAR transcriptional activity, and found commensurate induction in Tsc1 fl/fl and Tsc1 Δ/Δ BMDMs ( Fig. 2e ). Taken together, these findings indicate a selective defect in M2 polarization in Tsc1 Δ/Δ BMDMs that may not be due to defects in STAT6, PPARγ, or PPARδ expression or activity. mTORC1 activity attenuates IL-4-induced Akt activation The data above suggest that Tsc1 Δ/Δ BMDMs may not be able to activate some signals downstream of IL-4R. We turned our attention to IRS2/PI3K/Akt signalling, as this pathway is engaged by the IL-4R in parallel to the JAK/STAT6 pathway [29] , [30] . PI3K activation leads to increased activity of mTORC2, which phosphorylates Akt at S473 to activate the protein and promote membrane localization. In addition to S473, Akt is critically controlled by phosphorylation at T308, a step mediated by PDK1 ( Fig. 3a ). Thus we examined S473 and T308 phosphorylation as readouts of Akt activity, as well as phosphorylation of the downstream Akt targets FOXO1, PRAS40 and GSK-3 (ref. 31 ) ( Fig. 3a ). 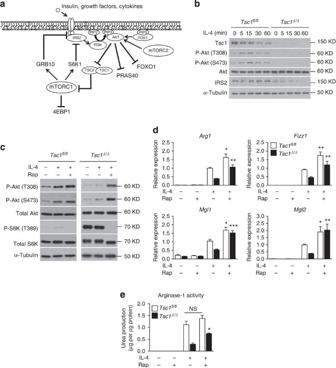Figure 3: Constitutive mTORC1 activity attenuates IL-4-induced Akt activation. (a) Overview of mTORC1 signalling downstream of IL-4, insulin and growth factors. Receptor activation engages the IRS/PI3K/Akt pathway. PI3K converts PIP2 to PIP3 thus recruiting PDK1 and Akt to the plasma membrane, enabling PDK1-mediated phosphorylation of Akt on T308. PI3K also activates mTORC2, which phosphorylates Akt on S473. Thus activated, Akt can phosphorylate downstream targets to regulate their activity. One consequence of Akt activation is increased mTORC1 activity, which feeds back to attenuate IRS2/PI3K/Akt signalling through multiple mechanisms, including reducing levels of IRS2 while increasing levels of GRB10. (b) Immunoblot analysis of lysates fromTsc1fl/flandTsc1Δ/ΔBMDMs stimulated with IL-4 for 5–60 min. (c) Immunoblot analysis of lysates fromTsc1fl/flandTsc1Δ/ΔBMDMs stimulated with IL-4 for 20 min in the presence or absence of rapamycin (20 nM, 1 h pretreatment). DMSO vehicle was used as control. (d) Expression of M2 genes inTsc1fl/flandTsc1Δ/ΔBMDMs after treatment with IL-4 for 15 h in the presence or absence of rapamycin (20 nM, 1 h pretreatment). (n=5). *P<0.05, **P<0.01, ***P<0.001 for IL-4 versus IL-4+rap. (e) Urea production normalized to total protein inTsc1fl/flandTsc1Δ/ΔBMDMs stimulated with IL-4 for 20 h in the presence or absence of rapamycin (20 nM, 1 h pretreatment). (n=5), *P<0.001. Graphs are shown as mean±s.e.m.Pvalues were determined using Student’st-tests. Figure 3: Constitutive mTORC1 activity attenuates IL-4-induced Akt activation. ( a ) Overview of mTORC1 signalling downstream of IL-4, insulin and growth factors. Receptor activation engages the IRS/PI3K/Akt pathway. PI3K converts PIP2 to PIP3 thus recruiting PDK1 and Akt to the plasma membrane, enabling PDK1-mediated phosphorylation of Akt on T308. PI3K also activates mTORC2, which phosphorylates Akt on S473. Thus activated, Akt can phosphorylate downstream targets to regulate their activity. One consequence of Akt activation is increased mTORC1 activity, which feeds back to attenuate IRS2/PI3K/Akt signalling through multiple mechanisms, including reducing levels of IRS2 while increasing levels of GRB10. ( b ) Immunoblot analysis of lysates from Tsc1 fl/fl and Tsc1 Δ/Δ BMDMs stimulated with IL-4 for 5–60 min. ( c ) Immunoblot analysis of lysates from Tsc1 fl/fl and Tsc1 Δ/Δ BMDMs stimulated with IL-4 for 20 min in the presence or absence of rapamycin (20 nM, 1 h pretreatment). DMSO vehicle was used as control. ( d ) Expression of M2 genes in Tsc1 fl/fl and Tsc1 Δ/Δ BMDMs after treatment with IL-4 for 15 h in the presence or absence of rapamycin (20 nM, 1 h pretreatment). ( n =5). * P <0.05, ** P <0.01, *** P <0.001 for IL-4 versus IL-4+rap. ( e ) Urea production normalized to total protein in Tsc1 fl/fl and Tsc1 Δ/Δ BMDMs stimulated with IL-4 for 20 h in the presence or absence of rapamycin (20 nM, 1 h pretreatment). ( n =5), * P <0.001. Graphs are shown as mean±s.e.m. P values were determined using Student’s t -tests. Full size image Interestingly, IL-4-stimulated Tsc1 Δ/Δ BMDMs displayed a striking attenuation in Akt signalling as indicated by reduced phosphorylation of Akt S473 and Akt T308 ( Fig. 3b ). Consistently, phosphorylation of the Akt targets FOXO1 and PRAS40 was diminished ( Supplementary Fig. S5a ). GSK-3 phosphorylation was not reduced ( Supplementary Fig. S5a ), perhaps because of its regulation by multiple inputs [32] , [33] , [34] , [35] . Importantly, diminished Akt signalling has been noted in TSC-deficient cells during stimulation with insulin and other growth factors [36] , [37] , [38] . Such reduction of Akt activity is due to mTORC1-mediated negative feedback that impinges on multiple targets, including but not limited to IRS1/2 degradation [39] , [40] and phosphorylation and stabilization of GRB10 (refs 41 , 42 ) ( Fig. 3a ). Although such mTORC1-mediated negative feedback is well defined for insulin signalling, little is known regarding its role in the regulation of cytokine signalling. Interestingly, we found that Tsc1 Δ/Δ BMDMs display reduced IRS2 levels in response to IL-4 treatment ( Fig. 3b ). This is likely to contribute to mTORC1-mediated attenuation of Akt signalling, as IRS2 has been implicated in Akt activation during IL-4 stimulation [29] . Increased levels of phosphorylated and total GRB10 ( Supplementary Fig. S5b ) may also have a role given that GRB10 inhibits signalling downstream of RTKs [43] , [44] , [45] . Thus increased mTORC1 activity in our model is likely to attenuate Akt signalling at least in part through IRS2 and GRB10. PDK1, the Akt T308 kinase, has constitutive kinase activity and is critically regulated by PIP3-mediated recruitment to the plasma membrane [46] , thus normal PDK1 activity in Tsc1 Δ/Δ BMDMs ( Supplementary Fig. S5c ) also supports our model that attenuated Akt signalling in Tsc1 Δ/Δ BMDMs occurs at a receptor proximal step upstream of PI3K-mediated PIP3 production ( Fig. 3a ). Finally, LPS-mediated Akt activation was diminished in Tsc1 Δ/Δ BMDMs, as evidenced by a defect in phosphorylation of Akt and the Akt target FOXO1 ( Supplementary Fig. S5d ). Collectively, these findings demonstrate that mTORC1-mediated negative feedback mechanisms converge to ultimately attenuate Akt signalling in Tsc1 Δ/Δ BMDMs. Having shown a defect in Akt activation in Tsc1 Δ/Δ BMDMs, we addressed a potential role in impaired M2 polarization. Previous studies have used rapamycin treatment to alleviate mTORC1-mediated negative feedback of Akt signalling and to interrogate the role of attenuated Akt activation in TSC-deficient models [36] , [37] , [38] . Accordingly, we found that rapamycin treatment of Tsc1 Δ/Δ BMDMs rescued IL-4-inducible Akt signalling ( Fig. 3c ). Importantly, such treatment restored induction of M2 genes Arg1 , Fizz1 and Mgl1/2 as well as Arginase activity ( Fig. 3d,e ). Together this suggests that deficient M2 polarization in Tsc1 Δ/Δ BMDMs may be due to mTORC1-mediated negative feedback of Akt signalling. We note that rapamycin treatment of control Tsc1 fl/fl BMDMs also modestly increased Akt signalling ( Fig. 3c ) as well as M2 responses ( Fig. 3d,e ), indicating that acute, signal-dependent activation of mTORC1 during IL-4 signalling can also feedback to inhibit Akt activation. Attenuated Akt signalling underlies aberrant polarization Our findings linking reduced Akt activation to impaired M2 polarization in Tsc1 Δ/Δ BMDMs ( Fig. 3b–e ) are interesting given that little is known regarding the role of Akt in this process. To address this directly, we treated WT BMDMs with MK-2206, an allosteric inhibitor of Akt. This led to a decrease in IL-4-inducible phosphorylation of Akt T308 and Akt S473 as well as the Akt target FOXO1, but did not affect STAT6 phosphorylation ( Fig. 4a ). Importantly, pretreatment with MK-2206 reduced IL-4-mediated induction of Arg1 , Fizz1 , Mgl2 and Mgl1 ( Fig. 4b ), as well as Arginase-1 activity ( Fig. 4c ). Similar effects were observed with the structurally distinct Akt inhibitor Akt VIII ( Supplementary Fig. S6a,b ), indicating the specificity of the inhibitors. These findings argue that Akt may have an important role in M2 polarization. Together with the data in Fig. 3 , they also support the idea that attenuated Akt signalling underpins defective M2 polarization in Tsc1 Δ/Δ BMDMs. 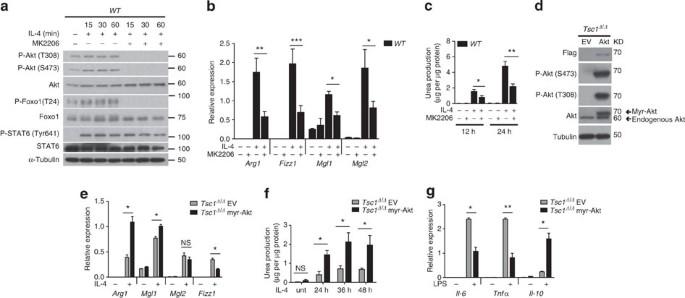Figure 4: Akt signalling is critical for polarization inTsc1Δ/ΔBMDMs. (a) Immunoblot analysis of WT BMDMs pretreated with MK-2206 for 1 h and treated with IL-4 for the indicated time points. (b,c) WT BMDMs were pretreated with MK-2206 or DMSO for 1 h before stimulation with IL-4 for 24 h and examination of (b) M2 gene expression (n=3) or (c) urea production (n=4). (d) Immunoblot analysis ofTsc1Δ/ΔBMDMs transduced with myr-flag-Akt or EV. (e,f) Myr-AktTsc1Δ/ΔBMDMs and EVTsc1Δ/ΔBMDMs were stimulated with IL-4 followed 24 h later by analysis of (e) M2 gene expression (n=4 representative experiments) or (f) urea production (n=3). (g) Cytokine gene expression in myr-AktTsc1Δ/ΔBMDMs and EVTsc1Δ/ΔBMDMs stimulated with LPS for 6 h (n=3). Graphs are shown as mean±s.e.m., *P<0.05, **P<0.01, ***P<0.001.Pvalues were determined using Student’st-tests. Figure 4: Akt signalling is critical for polarization in Tsc1 Δ/Δ BMDMs. ( a ) Immunoblot analysis of WT BMDMs pretreated with MK-2206 for 1 h and treated with IL-4 for the indicated time points. ( b , c ) WT BMDMs were pretreated with MK-2206 or DMSO for 1 h before stimulation with IL-4 for 24 h and examination of ( b ) M2 gene expression ( n =3) or ( c ) urea production ( n =4). ( d ) Immunoblot analysis of Tsc1 Δ/Δ BMDMs transduced with myr-flag-Akt or EV. ( e , f ) Myr-Akt Tsc1 Δ/Δ BMDMs and EV Tsc1 Δ/Δ BMDMs were stimulated with IL-4 followed 24 h later by analysis of ( e ) M2 gene expression ( n =4 representative experiments) or ( f ) urea production ( n =3). ( g ) Cytokine gene expression in myr-Akt Tsc1 Δ/Δ BMDMs and EV Tsc1 Δ/Δ BMDMs stimulated with LPS for 6 h ( n =3). Graphs are shown as mean±s.e.m., * P <0.05, ** P <0.01, *** P <0.001. P values were determined using Student’s t -tests. Full size image Next, we took a genetic approach to rescue Akt signalling in Tsc1 Δ/Δ BMDMs. As expected, retroviral transduction of Tsc1 Δ/Δ BMDMs with myristylated-Akt1 (myr-Akt) led to constitutive Akt signalling as indicated by high basal state P-Akt T308 and P-Akt S473 ( Fig. 4d ). Importantly, this was associated with increased induction of Arg1 and Mgl1 ( Fig. 4e ), as well as Arginase-1 activity ( Fig. 4f ), following IL-4 stimulation. Although ectopic expression of myr-Akt was insufficient to rescue Fizz1 and Mgl2 expression, this could be achieved in the context of rapamycin co-treatment ( Supplementary Fig. S6c ). Thus, myr-Akt may not fully recapitulate IL-4-inducible Akt activation; or alternatively, rescue of Akt signalling is not sufficient for restoring Mgl2 and Fizz1 expression, and some other consequence of constitutive mTORC1 activation is critically relieved by rapamycin treatment. Finally, to extend these studies to the proinflammatory responses, we examined myr-Akt expressing Tsc1 Δ/Δ BMDMs following LPS treatment. We observed significantly reduced expression of Il-6 and Tnf α but increased expression of Il-10 ( Fig. 4g and Supplementary Fig. S6d ). Deficient M2 polarization in Tsc1 Δ/Δ mice Finally, we asked whether TSC1 deficiency would impair M2 polarization in vivo . We used intraperitoneal (IP) injection of an IL-4/IL-4 antibody complex to elicit IL-4-dependent recruitment and in situ proliferation of M2 macrophages [47] in Tsc1 fl/fl and Tsc1 Δ/Δ mice. Strikingly, induction of most M2 genes was decreased in peritoneal exudate cells (PECs) from Tsc1 Δ/Δ mice ( Fig. 5a ). To corroborate these findings, we used a model of chitin administration that triggers IL-4-dependent recruitment and polarization of M2 macrophages [48] , [49] . We observed a near universal reduction of M2 gene expression in Tsc1 Δ/Δ PECs ( Fig. 5b ), similar to the IL-4 injection. Collectively, the findings support our model that constitutive mTORC1 activity can attenuate macrophage M2 polarization in vivo . 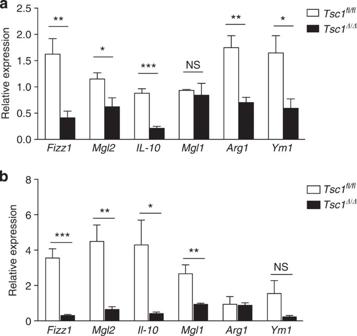Figure 5: M2 polarization inTsc1Δ/Δmice is impairedin vivo. (a) M2 gene expression in PECs fromTsc1Δ/ΔandTsc1fl/flmice 4 days post IP injection with IL-4c on days 0 and 2 (n=4 mice per genotype). (b) M2 gene expression in PECs from maleTsc1Δ/ΔandTsc1fl/flmice 48 h post IP injection with chitin (n=5 mice per genotype). Data shown as mean±s.e.m., *P<0.05, **P<0.01, ***P<0.001.Pvalues were determined using Student’st-tests. Figure 5: M2 polarization in Tsc1 Δ/Δ mice is impaired in vivo . ( a ) M2 gene expression in PECs from Tsc1 Δ/Δ and Tsc1 fl/fl mice 4 days post IP injection with IL-4c on days 0 and 2 ( n =4 mice per genotype). ( b ) M2 gene expression in PECs from male Tsc1 Δ/Δ and Tsc1 fl/fl mice 48 h post IP injection with chitin ( n =5 mice per genotype). Data shown as mean±s.e.m., * P <0.05, ** P <0.01, *** P <0.001. P values were determined using Student’s t -tests. Full size image In this study, we use a novel model of myeloid-specific Tsc1 deletion and constitutive mTORC1 activity to elucidate mTORC1 function in macrophages. We found that Tsc1 Δ/Δ BMDMs have enhanced proinflammatory cytokine production while IL-10 secretion is reduced, in line with a recent analysis of Tsc1 Δ/Δ BMDMs [17] . Other studies reached conflicting conclusions, using small hairpin RNA knockdown in monocytes and dendritic cells [50] , [51] . Extending the analysis of mTORC1 function in macrophages, we showed that Tsc1 Δ/Δ BMDMs are impaired in M2 polarization, expressing reduced levels of key M2 markers such as Arg1 , Fizz1 , Mgl1 , Mgl2 , Ym1 and Pgc-1β ( Fig. 1d ). Interestingly, the defect in M2 activation seems to be selective, as induction of PPARγ- and some PPARγ-dependent genes (for example, Cd36 and Fabp4 ) occur normally ( Fig. 2c,d ). In addition, we find that Tsc1 Δ/Δ BMDMs have diminished levels of Arginase-1 activity and fatty acid oxidation, hallmark features of M2 macrophages ( Fig. 1e,f ). This suggests that mTORC1 may couple regulation of fatty acid oxidation to control macrophage polarization, consistent with the emerging view that macrophage cellular metabolism is closely linked to activation status [3] , [8] , [52] . Finally, we use models of IL-4 and chitin injection to show that constitutive mTORC1 activity in myeloid lineage cells results in broad defects in M2 polarization in vivo ( Fig. 5 ). Normal activation of known regulators of M2 polarization, including STAT6, PPARγ and PPARδ ( Fig. 2 ), suggests that impaired M2 polarization in Tsc1 Δ/Δ BMDMs may be due to block of a parallel signalling pathway. In addition to the JAK/STAT6 pathway, IL-4R signalling engages IRS2/PI3K signalling in parallel to mediate Akt activation [29] , [30] . Although STAT6 is indispensable for M2 polarization [1] , [53] , the role of Akt signalling has not been well characterized. Our findings suggest a critical role for mTORC1-mediated feedback inhibition of Akt signalling in Tsc1 Δ/Δ BMDMs. In support of this, Tsc1 Δ/Δ BMDMs display decreased IL-4-inducible Akt activation, as indicated by diminished P-Akt T308 and P-Akt S473 ( Fig. 3b ) and phosphorylation of the Akt targets FOXO1 and PRAS40 ( Supplementary Fig. S5a ). Importantly, rapamycin treatment ( Fig. 3c–e ) and ectopic expression of myr-Akt ( Fig. 4d–f , Supplementary Fig. S6c ) restore Akt activation simultaneous with rescue of M2 gene expression and Arginase activity. We suggest that decreased IRS2 ( Fig. 3b ) but increased GRB10 ( Supplementary Fig. S5b ) levels may contribute to mTORC1-mediated attenuation of Akt signalling, as IRS2 has been implicated in IL-4R signalling [54] , while GRB10 downregulates signalling downstream of RTKs [43] . Although other negative feedback mechanisms have been described in insulin signalling [40] , [55] and may exist in our setting, they act synergistically and ultimately converge to attenuate Akt activation. Finally, we believe that feedback inhibition to Akt may also underlie the enhanced responsiveness of Tsc1 Δ/Δ BMDMs to LPS stimulation. Although we have not extensively characterized the underlying mechanism(s) in this context, Akt activation in Tsc1 Δ/Δ BMDMs is diminished following LPS signalling ( Supplementary Fig. S5d ), and its rescue with myr-Akt expression reduces the exaggerated responses ( Fig. 4g ). Importantly, control of M2 polarization by Akt signalling is likely to extend beyond our genetic model to other settings, as pharmacological inhibition of Akt impairs M2 activation in wild-type BMDMs ( Fig. 4b,c , Supplementary Fig. S6a,b ). Moreover, rapamycin treatment of control BMDMs modestly increases Akt signalling and M2 responses ( Fig. 3c–e ). Thus our findings reveal a largely unappreciated role for Akt in synergizing with the STAT6 pathway to regulate full M2 polarization ( Fig. 6a ). Whether Akt promotes or inhibits inflammation downstream of LPS signalling is not entirely clear [56] , but at least in Tsc1 Δ/Δ BMDMs, simultaneous mTORC1 activation and Akt attenuation lead to enhanced proinflammatory responses that can be rescued by restoring Akt signalling ( Fig. 4g ). The relevant Akt targets that regulate macrophage polarization are not well defined, but could include FOXO1 and CEBPβ [57] , [58] . Interestingly, macrophages deficient in Rictor, a subunit of the mTORC2 complex that phosphorylates Akt on S473, were deficient in some but not all Akt-dependent activities ( Supplementary Fig. S7a ) consistent with previous models of mTORC2 deficiency [59] , [60] but polarized normally to the M2 phenotype ( Supplementary Fig. S7b,c ), and could serve as a plausible model to identify the relevant Akt targets controlling M2 activation. 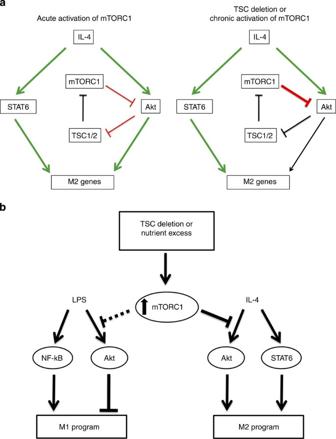Figure 6: Proposed model for how mTORC1 activity controls macrophage polarization. (a) Physiological induction of the Akt-mTORC1 signalling loop by IL-4 stimulation (left) allows for transient, inducible activation of the pathway, and enables Akt to synergize with the JAK/STAT pathway for M2 polarization. mTORC1 activity is also regulated by nutrient availability (not shown here), so such wiring of the signalling pathway may allow calibration of M2 activation to metabolic status (left). In contrast, constitutive or aberrant mTORC1 activation corrupts this signalling pathway and modulation of macrophage activation by metabolic inputs (right). (Green=activation; red=inhibition; black=attenuated) (b) Constitutive or aberrant activation of mTORC1 impairs the ability of macrophages to respond appropriately to polarizing stimuli. A critical mediator of this process is Akt, whose activity is downregulated by increased mTORC1 activity. Figure 6: Proposed model for how mTORC1 activity controls macrophage polarization. ( a ) Physiological induction of the Akt-mTORC1 signalling loop by IL-4 stimulation (left) allows for transient, inducible activation of the pathway, and enables Akt to synergize with the JAK/STAT pathway for M2 polarization. mTORC1 activity is also regulated by nutrient availability (not shown here), so such wiring of the signalling pathway may allow calibration of M2 activation to metabolic status (left). In contrast, constitutive or aberrant mTORC1 activation corrupts this signalling pathway and modulation of macrophage activation by metabolic inputs (right). (Green=activation; red=inhibition; black=attenuated) ( b ) Constitutive or aberrant activation of mTORC1 impairs the ability of macrophages to respond appropriately to polarizing stimuli. A critical mediator of this process is Akt, whose activity is downregulated by increased mTORC1 activity. Full size image Our studies indicate the existence of a mTORC1–Akt regulatory loop in the IL-4 signalling pathway that parallels that of the insulin pathway. In the latter, a feedback loop between mTORC1 and Akt—in which receptor engagement of the IRS/PI3K/Akt pathway leads to mTORC1 activation that feeds back to attenuate Akt signalling—is critical for transient, signal-dependent activation of these two signalling modules ( Fig. 3a ). Similarly, activation of the IRS2/PI3K/Akt pathway by IL-4 mediates mTORC1 activation ( Fig. 1a , Supplementary Fig. S8 ) and as shown here, results in feedback inhibition of Akt signalling ( Fig. 3a–c , Fig. 6a ). Importantly, mTORC1 activity is critically modulated by nutrient/energy availability [61] , thus we propose that integration of the mTORC1–Akt regulatory loop into the IL-4 signalling pathway may allow macrophages to calibrate their activation and function to metabolic status and nutrient availability ( Fig. 6a ). In contrast, this regulatory circuitry is disrupted by constitutive or aberrant activation of mTORC1, as occurs during nutrient excess or in our genetic model. As a consequence, induction of M2 polarization by the synergistic interactions of the Akt and JAK/STAT pathways is impaired ( Fig. 6a,b ). Conversely, elevated mTORC1 activity and consequent downregulation of Akt signalling may facilitate increased responses to LPS stimulation ( Fig. 6b ). Finally, we note that such ‘hard-wiring’ of mTORC1–Akt signalling to cytokine signalling could have relevance to other immunological contexts, given that many cytokines that regulate immune cell function engage the Akt pathway (and presumably also mTORC1). In conclusion, our study highlights a key role of the mTORC1 pathway in control of macrophage polarization. Such control is likely to be of particular relevance for adipose tissue macrophages (ATMs). In the lean state, ATMs with a M2 phenotype maintain an anti-inflammatory environment and adipocyte insulin sensitivity, whereas in obesity, ATMs with a M1 phenotype produce inflammatory cytokines and promote insulin resistance and metabolic dysfunction. We propose that nutrient sensing by mTORC1 may directly regulate the pathophysiological switch of ATMs during obesity, extending the current model for regulation of the pathophysiological M2 to M1 switch [62] . Indeed, given that macrophages are critical orchestrators of diverse physiological responses, regulation of macrophage activation by the mTOR pathway may have profound consequences in many settings, including helminth infection, inflammation, allergy and tissue repair. BMDMs Briefly, femurs were removed from mice after CO2 euthanasia, and cells were liberated using a mortar and pestle. For macrophage differentiation, bone marrow-derived cells were plated in Petri dishes with 1640 RPMI media (10% FCS, penicillin/streptomycin, 2 mM L -Glutamine) supplemented with MCSF-containing L929 cell supernatant for 7 days. MCSF-differentiated macrophages were harvested and plated in tissue culture dishes for subsequent experiments. For M1-like activation, 0.5-0.7 × 10 6 BMDMs were plated in 12-well tissue culture dishes and treated with 10 ng ml −1 LPS (Invivogen). For M2(a) polarization, cells were treated with 10 ng ml −1 IL-4 (Peprotech). For M2(b) polarization, cells were treated with 10 ng ml −1 IL-10 (Peprotech). For M2b polarization, cells were treated simultaneously with 10 ng ml −1 LPS (Invivogen) and either unopsonized sheep red blood cells (SRBC) (Lampire biological laboratories) or SRBCs opsonized with 1:400 anti-SRBC immunoglobulin G (cat# 55806 MP Biomedicals). Mice To generate mice with targeted deletion of Tsc1 in myeloid lineage cells, mice with flanking loxP Tsc1 alleles ( Tsc1 fl/fl ) were crossed to LysozymeM Cre transgenic mice, both on a B6 background [38] , [63] . Cre-recombinase activity results in deletion of exons 17 and 18 of Tsc1 , generating a null allele [64] . Male mice aged 12 weeks were used for in vivo chitin administration and male mice aged 6–8 weeks were used for in vivo IL-4 administration. For Rictor deletion in vivo , tamoxifen (VWR) was suspended in sunflower seed oil (VWR) at 10 mg ml −1 , and 200 μl per 25 g body weight was injected into 10-week old Rictor fl/fl and Rictor fl/fl UbiquitinC- CreERT2 mice once daily for 7 days [65] . Bone marrow from such mice was used to generate Rictor-deficient macrophages. Mice were maintained at Harvard Medical School and Massachusetts Institute of Technology, and all procedures were performed in accordance with the guidelines set forth by the Institutional Animal Care and Use Committees at each institution. Immunoblotting For protein sample preparation, cells were washed twice with cold phosphate-buffered saline (PBS) following stimulation and lysed in 1% NP-40 buffer with EDTA-free protease inhibitor tablets (Roche Diagnostics) and phosphatase inhibitors. Protein concentration in lysates was determined using the Bradford method. Equal amounts of protein were loaded onto SDS–PAGE gels and subsequently transferred to polyvinylidene difluoride membranes for immunoblotting with primary antibodies as indicated. Full blots of all immunoblots shown in the main article are included in Supplementary Fig. S9 . Antibodies and reagents Primary antibodies were purchased from Cell Signaling (all at 1:1,000 dilution in 5% bovine serum albumin (BSA)), except for the following: α- Tubulin (Sigma, 1:5,000), β-Actin (Sigma, 1:2,000), Flag-M2 (Sigma, 1:1,000) and PPARγ (Santa Cruz E-8, 1:1,000) and PPARδ (Santa Cruz, 1:250). For flow cytometry, antibodies used were CD11b-PE (BD Biosciences) and F4/80-FITC (BioLegend). Inhibitors were used as follows: MK-2206 1 μM (Selleck), Akt VIII 10 μM (Enzo), rapamycin 20 nM (LC Laboratories), Troglitazone 1 μM (Cayman) and GW501516 100 μM (Enzo). Arginase assays Arginase assay was described previously [66] . Briefly, 0.5 × 10 6 cells per well in 12-well plates were stimulated with IL-4 for 12–48 h. Cells were lysed in 0.1% TritonX-100 lysis buffer with protease inhibitors. Lysates with equal amounts of protein were incubated with 500 mM L -Arginine for 45 min at 37 °C, followed by acid stop solution. The degradation of L -arginine to urea was measured by adding 9% isonitrosopropiophenone in 100% ethanol. Absorbance was read at 540 nm in a microplate reader. All samples were read in triplicate. Fatty acid oxidation BMDMs were plated 0.7 × 10 6 cells per well in 12-well tissue culture dishes in complete RPMI and stimulated with IL-4 for 36 h. After stimulation, cells were washed with PBS and loaded with low-glucose Dulbecco's Modified Eagle Medium +2% fatty acid-free BSA (Lampire Biologicals) for 30 min at 37 °C. After 30 min, cells were washed with PBS and given 3 H-labelled palmitic acid (2 μCi per well, MP Biomedicals) in low-glucose Dulbecco's Modified Eagle Medium, with 2% fatty acid-free BSA and 0.2 mM unlabelled oleic acid (Sigma). After 4 h, 100 μl of media was collected and the isolation of 3 H2O was performed using trichloroacetic acid followed by chloroform–methanol extraction. The water-soluble fraction was collected in 5 ml of EcoLume (MP Biomedicals) scintillation fluid and counted for 5 min using a Beckman LS6500 scintillation counter. Cells were lysed in 500 μl of 0.1N NaOH and total protein was determined using the Bradford method. Background 3 H was subtracted from the c.p.m. (counts per minute) value and all samples were normalized to a milligram of total protein. All samples were performed in duplicate. Myr-Akt-transduction To make retrovirus particles, 293T cells were co-transfected with pBabe empty vector Puro or pBabe Puro Myr Flag Human-Akt1 purchased from Addgene (plasmid 15294) along with pCL-Eco (Imgenex #10045P) using Lipofectamine 2000 (Invitrogen). Transfected 293T media was changed the next day and placed at 32 °C. Viral supernatant was collected on day 2 and day 3 post transfection. Fresh bone marrow was plated on the same day as transfection above and transduced with media containing viral supernatant (50% viral supernatant containing pBabe empty vector or pBabe Puro Myr Flag Human-Akt1, 40% RPMI complete media, and 10% CMG media) on day 2 and day 3 and selected using 4 μg ml −1 puromycin on days 4–7. ELISA Cytokine concentration was determined using for IL-10, TNFα and IL-6 using ELISA kits purchased from BioLegend. Briefly, experimental supernatants were collected and centrifuged at 3,000 g per 5 min. Supernatants were analysed in duplicate per manufacturers protocol. Chromatin immunoprecipitation For STAT6 ChIP, BMDMS (5 × 10 6 ) were plated in 6 cm tissue culture plates and stimulated for 2 h with 10 ng ml −1 IL-4. Cells were subsequently fixed with 1% formaldehyde for 10 min at room temperature. Formaldehyde was quenched with glycine. After collecting cells, lysis was performed using 500 μl of SDS buffer (1% SDS, 10 mM EDTA, 50 mM Tris-Cl pH 8) plus protease and phosphatase inhibitors. Cells were subsequently sonicated for 3 min on ice with 1-s pulses using a Misonix 4000 sonicator to shear chromatin. Following sonication, samples were diluted to 3 ml with ChIP dilution buffer (0.01% SDS, 1.1% Triton X-100, 1.2 mM EDTA, 16.7 mM Tris-Cl pH 8, 167 mM NaCl) and precleared for 1 h at 4 °C with protein A salmon sperm/agarose beads (Millipore). Precleared chromatin was split into 400 μl aliquots for IP with either 5 μg of STAT6 (M-20 ChIP grade, Santa Cruz) or for no antibody control overnight at 4 °C. IPs were incubated with protein A salmon sperm/agarose beads (Millipore) the following day for 3 h at 4 °C. After 3 h, beads were spun down and ~10% of chromatin was taken for input and processed in parallel to IP samples. Antibody bead complexes were then washed with low salt (0.1% SDS, 1% Triton X-100, 2 mM EDTA, 20 mM Tris-Cl pH 8, 150 mM NaCl), high salt (0.1% SDS, 1% Triton X-100, 2 mM EDTA, 20 mM Tris-Cl pH 8, 500 mM NaCl) and lithium chloride (0.25 M LiCl, 1% deoxycholic acid, 1% NP-40, 1 mM EDTA, 10 mM Tris-Cl pH 8) buffers followed by two washes with TE buffer. Chromatin–antibody complexes were eluted with elution buffer (1% SDS±0.1 M sodium bicarbonate) and crosslinks were reversed using sodium chloride and incubation at 60 °C for 4 h. Samples were then incubated 1 h with proteinase K (Roche) at 60 °C. DNA was purified using PCR purification columns (Qiagen) and used for quantitative PCR with primers generated to the Arg1 promoter region. Fold enrichment was calculated as ChIP signals divided by no antibody control and normalized to input. Quantitative PCR To measure gene expression in BMDMs and PECs, RNA was isolated using RNA Bee (Tel-Test) per manufacturers protocol and used to make cDNA using High Capacity cDNA Reverse Transcription Kit (Applied Biosystems). A Bio-Rad C1000 Thermocycler was used to analyse the samples under the following conditions: 95 °C (5 min), 50 cycles of 95 °C (10 s), 60 °C (10 s), and 72 °C (20 s). Reaction mixture consisted of 4 μl cDNA, 1.5 μl 3 μM primers for each gene used in the study (F+R), 2 μl H2O, and 7.5 μl 2 × SYBR green (Bio-Rad). Samples from BMDMs were normalized to hypoxanthine phosphoribosyltransferase and samples from PECs were normalized to the macrophage marker CD68. Data were analysed by means of the CFX Manger Software (Bio-Rad) using the delta/delta CT method. Sequences for all qPCR primers are shown in Supplementary Table S1 . Chitin administration Chitin (Sigma) was prepared as previously described [48] . Briefly, chitin was washed three times with PBS and then sonicated (Misonix Sonicator 4000) for 30 min on ice. The dissolved chitin was filtered and diluted with PBS to 4 μg ml −1 . 800 ng chitin dissolved in 200 μl of PBS was injected IP and PECs were collected 48 h post injection. IL-4 complex administration Long acting IL-4 complex (IL-4c) was prepared as previously described [47] . Briefly, IL-4 (Peprotech) was suspended at a concentration of 500 μg ml −1 and mixed with anti-mouse IL-4 (BioXcell clone 11b11) at a molar ratio of 2:1 (weight 1:5) and incubated 1–2 min at room temperature. IL-4c was suspended in normal saline to a concentration of 25 μg ml −1 IL-4 and 125 μg ml −1 of 11b11. Each mouse was injected IP with 200 μl of IL-4c (5 μg IL-4 and 25 μg 11b11) on day 0 and 2, and PECs were collected on day 4. Dual luciferase assays BMDMs were electroporated using Amaxa nucleofector and mouse macrophage nucleofector kit (Lonza) with PPAR-Firefly luciferase plasmid (C.H. Lee, Harvard School of Public Health) or STAT6-Firefly luciferase (purchased from Addgene-plasmid #35554) along with Renilla–Luciferase plasmid as a transfection control. The PPAR- Firefly luciferase plasmid consists of three copies of the Acox1 PPAR response element [67] upstream of an SV40 minimal promoter. BMDMs were treated with IL-4 and/or troglitazone 4 h post electroporation for 24 h. Cell lysates were collected and analysed using the Promega Dual-Luciferase Reporter Assay System. Statistical analysis Statistical analysis was carried out using Prism (GraphPad) software. The student’s t -test was used to determine statistical significance, defined as P <0.05. How to cite this article: Byles, V. et al. The TSC-mTOR pathway regulates macrophage polarization. Nat. Commun. 4:2834 doi: 10.1038/ncomms3834 (2013).